Formation and maintenance of neuronal assemblies through synaptic plasticity The architecture of cortex is flexible, permitting neuronal networks to store recent sensory experiences as specific synaptic connectivity patterns. However, it is unclear how these patterns are maintained in the face of the high spike time variability associated with cortex. Here we demonstrate, using a large-scale cortical network model, that realistic synaptic plasticity rules coupled with homeostatic mechanisms lead to the formation of neuronal assemblies that reflect previously experienced stimuli. Further, reverberation of past evoked states in spontaneous spiking activity stabilizes, rather than erases, this learned architecture. Spontaneous and evoked spiking activity contains a signature of learned assembly structures, leading to testable predictions about the effect of recent sensory experience on spike train statistics. Our work outlines requirements for synaptic plasticity rules capable of modifying spontaneous dynamics and shows that this modification is beneficial for stability of learned network architectures. Cortical neurons undergo complex and variable activity fluctuations during spontaneous dynamics [1] , [2] , [3] , but how this activity relates to functional processing is poorly understood. Several studies have observed spontaneous reactivation of evoked activity patterns without stimulus application [4] , [5] , [6] , [7] . The spiking variability of pairs of neurons due to shared network architecture increases with the overlap in their stimulus preferences [8] , [9] , [10] . Together, these observations suggest spontaneous dynamics are related to previously experienced stimuli. This is likely due to synaptic plasticity that reorganizes networks to reflect past activation patterns [11] , [12] , [13] . This view is consistent with studies showing that connections between similarly tuned visual cortical neurons are more probable [14] and that this specificity emerges after eye opening [15] . To address the mechanisms behind these observations, realistic models of both spontaneous dynamics and plasticity are needed. Model networks with balanced excitation and inhibition have addressed the first concern, reproducing the high variability of spontaneous cortical dynamics [16] , [17] , [18] . Many prior models of plasticity in spiking neuronal networks have neglected this balance, modelling few synapses per neuron [19] or normalizing network firing rates rather than modelling inhibition [20] . Conversely, work in balanced attractor circuits has lacked realistic plasticity mechanisms [21] , [22] . This is in part due to the fact that previous attempts to embed spike timing-dependent plasticity (STDP) in balanced networks have led to pathological behaviour [23] . Recently, detailed STDP models have been proposed [24] , [25] , [26] , but studies so far have been restricted to small or homogeneous networks. One central difficulty is that spontaneous activity in plastic networks can destabilize learned network architectures, especially if spontaneous fluctuations are similar in magnitude to evoked responses [2] . Many models do not study this possibility or assume plasticity is inactivated after learning [22] , [25] . Prior theoretical studies have suggested that reactivation of trained patterns can prevent degradation of learned architectures [27] , [28] , but have not done so in spiking networks with spontaneous activity. Thus, it is unclear how the plasticity mechanisms that ensure the stability of learned network architectures coexist with the fluctuations that define spontaneous cortical dynamics. We study balanced networks with realistic STDP [25] , showing that stimulus application leads to interconnected neuronal assemblies. After training, spontaneous dynamics reflect experienced stimuli, with transient reactivations of previously trained assemblies. These dynamics depend on maintenance of the learned connectivity by homeostatic mechanisms [29] , [30] . Furthermore, we show that cortical trial-to-trial variability is sufficient for spontaneous assembly reactivation, promoting stability of learned patterns. Our model is the first to demonstrate stable modification of spontaneous dynamics in balanced networks through realistic STDP mechanisms. It also suggests that the interaction between spontaneous dynamics and STDP plays an important role in memory stability. Instability of Hebbian STDP without homeostasis While many studies have investigated the dynamics of balanced networks with fixed connection weights, few have investigated the case of plastic synapses. We simulated a model cortical network of excitatory and inhibitory neurons, supplemented with plasticity rules that modified connections onto excitatory neurons (see Methods). The network was composed of 4,000 adaptive exponential integrate-and-fire excitatory neurons and 1,000 integrate-and-fire inhibitory neurons [31] , [32] coupled randomly with a connection probability of 0.2. Excitatory-to-excitatory synapses were governed by a voltage-based STDP rule [25] ( Fig. 1a , top). The STDP rule captured the dependence of long-term depression and potentiation on firing rate [33] ( Fig. 1a , bottom), so that neurons that exhibited correlated rate fluctuations tended to recruit long-term potentiation. 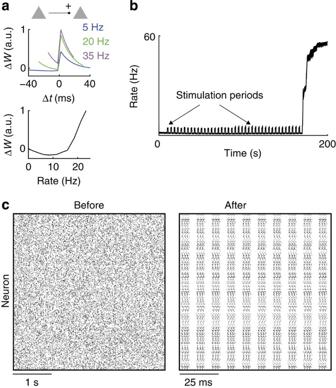Figure 1: Pathological activity after training in a network without homeostasis. (a) STDP curve for different pairing frequencies (top) and weight change as a function of firing rate assuming both neurons fire as Poisson processes with the same rate (bottom). (b) Average excitatory firing rate as a function of time. (c) Excitatory neuron spike rasters before training and after 200 s of training. After ~200 s, the network dynamics settle into high-frequency oscillations. Figure 1: Pathological activity after training in a network without homeostasis. ( a ) STDP curve for different pairing frequencies (top) and weight change as a function of firing rate assuming both neurons fire as Poisson processes with the same rate (bottom). ( b ) Average excitatory firing rate as a function of time. ( c ) Excitatory neuron spike rasters before training and after 200 s of training. After ~200 s, the network dynamics settle into high-frequency oscillations. Full size image We investigated whether external stimuli could modify the network’s structure and dynamics through STDP. We began with a network with a homogeneous weight structure. The network exhibited irregular and asynchronous firing due to a balance between excitatory and inhibitory currents [16] , [17] . Neuronal assemblies did not form spontaneously, as the uniformly low firing rates tended to recruit depression ( Supplementary Fig. 1 ). To investigate how this connectivity could be modified by the application of external stimuli, we defined a set of 20 stimulus patterns, which when active corresponded to an increased excitatory drive to neurons targeted by that pattern. Neurons were targeted by each pattern with a probability of 0.05. Consequently, the number of stimuli targeting each neuron was binomially distributed. Approximately 36% of neurons were not targeted, 38% were targeted by one stimulus and 26% were targeted by multiple stimuli. For each stimulus i =1, 2, …, 20, we refer to those neurons targeted by the stimulus as neuronal assembly i . Stimuli were presented sequentially in repeated presentation blocks. Each stimulus presentation increased the external drive to targeted neurons by 8 kHz, which may be interpreted as an increase in the firing rate of 1,000 presynaptic neurons by 8 Hz each, on average. Stimulus presentations lasted 1 s, with 3-s gaps between stimuli (see Methods). Stimuli recruited increased firing rates in subsets of the network ( Fig. 1b ). However, as has been reported in previous studies of balanced networks with STDP [23] , [34] , after a few tens of stimulus applications, the network firing rate increased abruptly ( Fig. 1b ) and exhibited high frequency oscillations ( Fig. 1c ) that reflected a loss of stability of the asynchronous balanced state. These dynamics were due to runaway positive feedback of Hebbian STDP during training [35] . Indeed, such instability has precluded the development of realistic models of stimulus-evoked plasticity in such systems [23] . Our study investigates homeostatic mechanisms for synaptic plasticity [34] , [35] , which regulate network activity, preventing this instability and producing spontaneous dynamics consistent with experimental data from cortex. Formation of neuronal assemblies We implemented a recently proposed symmetric Hebbian STDP rule that acted on inhibitory to excitatory synapses [30] ( Fig. 2a ). This inhibitory synaptic plasticity (iSTDP) controlled the firing rate of excitatory neurons, as frequently firing neurons recruited more inhibition, while low-firing rate neurons recruited less inhibition [30] We also normalized the total excitatory conductance onto any neuron [36] , [37] , thus imposing competition between synapses (note that our results hold for a variety of soft normalization time scales; Supplementary Fig. 2 ). 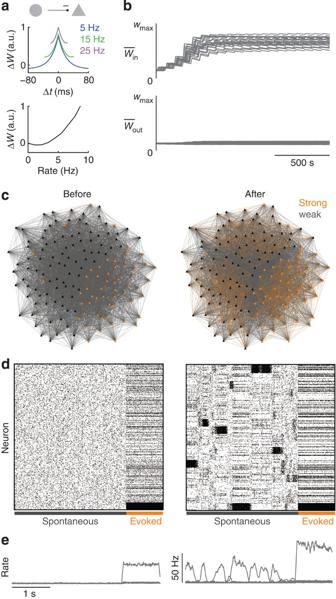Figure 2: Modification of weights and spontaneous activity by training in a network with homeostasis. (a) Inhibitory STDP curve for different pairing frequencies (top) and weight change as a function of firing rate assuming both neurons fire as Poisson processes with the same rate (bottom). (b) Average synaptic weightfor synapses between neurons within an assembly (top) andfor synapses between neurons in different assemblies (bottom). (c) Graph showing connection strength between neuron pairs for 50 neurons sampled from three assemblies before (left) and after (right) training. Orange lines correspond to strong excitatory connections. Neurons in the same assembly are placed nearby one another. Coloured nodes indicate neurons targeted by stimulus 1. Due to assembly membership overlap, some of these targeted neurons are also in the assemblies corresponding to stimuli 2 and 3. (d) Excitatory neuron spike rasters before and after training. Adjacent rows in the raster correspond to neurons in the same assembly. Some rows are repeated since neurons can belong to multiple assemblies. Neurons not belonging to assemblies are not shown. (e) Average firing rate for neurons in each assembly, corresponding to the activity ind. Figure 2: Modification of weights and spontaneous activity by training in a network with homeostasis. ( a ) Inhibitory STDP curve for different pairing frequencies (top) and weight change as a function of firing rate assuming both neurons fire as Poisson processes with the same rate (bottom). ( b ) Average synaptic weight for synapses between neurons within an assembly (top) and for synapses between neurons in different assemblies (bottom). ( c ) Graph showing connection strength between neuron pairs for 50 neurons sampled from three assemblies before (left) and after (right) training. Orange lines correspond to strong excitatory connections. Neurons in the same assembly are placed nearby one another. Coloured nodes indicate neurons targeted by stimulus 1. Due to assembly membership overlap, some of these targeted neurons are also in the assemblies corresponding to stimuli 2 and 3. ( d ) Excitatory neuron spike rasters before and after training. Adjacent rows in the raster correspond to neurons in the same assembly. Some rows are repeated since neurons can belong to multiple assemblies. Neurons not belonging to assemblies are not shown. ( e ) Average firing rate for neurons in each assembly, corresponding to the activity in d . Full size image We recorded , the average synaptic strength of connections in each of the 20 neuronal assemblies. During the training period, this quantity increased as stimuli were presented, until synapses between neurons in the same assembly were strongly potentiated ( Fig. 2b,c ). Due to the normalization of excitatory conductance, decreased slightly on average ( Fig. 2b , bottom). Despite this reorganization, the average excitatory firing rate after training did not diverge, stabilizing at ~1.7 Hz ( Supplementary Fig. 3 ). Besides modifying synaptic weights, training also changed the network’s spontaneous dynamics. The clustered excitatory connectivity led to transient activations of previously stimulated neuronal assemblies ( Fig. 2d,e ; Supplementary Movie 1 ). These high-firing rate activations occurred over a time scale of hundreds of milliseconds. However, due to infrequent activations, the time-averaged firing rates of individual neurons remained low, consistent with recordings from spontaneous cortex [2] , [3] . We conclude that the network reorganizes its connections in response to stimulus presentation, and that this reorganization substantially modifies spontaneous dynamics to reflect prior stimuli. We refer to these new dynamics as structured spontaneous activity, in contrast to the uncorrelated activity in the homogeneously connected network. Effects of homeostatic inhibitory plasticity Under the iSTDP rule, inhibitory synapses were potentiated when the postsynaptic excitatory neuron fired above a target firing rate and depressed otherwise ( Fig. 2a ). As a result, the rule homeostatically regulated the distribution of excitatory firing rates in the network towards this target value. We next investigate how this mechanism permits stable formation of assemblies. A frequently encountered challenge in networks with multiple stable states is winner-take-all dynamics, in which a single stable state, typically characterized by a specific subset of neuronal subpopulations with high firing rates, is dominant [18] . In such networks, high-firing rate subpopulations suppress the rest of the network, preventing other neurons from responding to inputs or exhibiting strong spontaneous fluctuations. In general, fine-tuning of parameters is needed to avoid these pathological states [36] . To robustly prevent winner-take-all dynamics, a mechanism by which high-firing rate neurons are suppressed is necessary. The iSTDP rule satisfies this requirement. Indeed, after training, certain assemblies received more inhibition than others ( Fig. 3b ). This heterogeneity prevented winner-take-all dynamics during training. Blocking iSTDP led to less potentiation for stimulated assemblies ( Fig. 3c ) and spontaneous activity in which only a single assembly exhibited high firing rates ( Fig. 3d ). Thus, we conclude iSTDP is necessary to prevent winner-take-all dynamics that would eventually lead to a degradation of connectivity between suppressed assemblies. 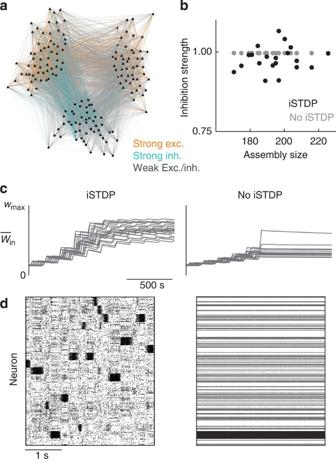Figure 3: Effects of inhibitory STDP. (a) Schematic showing connections between two assemblies and inhibitory neurons. One strongly connected and one weakly connected assembly is shown. Orange lines correspond to strong excitatory connections and blue lines to strong inhibitory connections. (b) Average inhibitory connection strength onto assemblies of different sizes for networks with and without iSTDP. (c) Average connection strength within assembliesduring training for networks with (left) and without (right) iSTDP. (d) Spike rasters during spontaneous activity for networks with (left) and without (right) iSTDP. Figure 3: Effects of inhibitory STDP. ( a ) Schematic showing connections between two assemblies and inhibitory neurons. One strongly connected and one weakly connected assembly is shown. Orange lines correspond to strong excitatory connections and blue lines to strong inhibitory connections. ( b ) Average inhibitory connection strength onto assemblies of different sizes for networks with and without iSTDP. ( c ) Average connection strength within assemblies during training for networks with (left) and without (right) iSTDP. ( d ) Spike rasters during spontaneous activity for networks with (left) and without (right) iSTDP. Full size image Stability of learned connectivity We next examined the stability of the network architecture during structured spontaneous activity. Many studies have examined how different synaptic dynamics can affect the stability of learned connectivity in the face of random spontaneous firing, employing models that include, for example, cascades of synaptic states [38] or metaplasticity [39] . We took a complementary approach, asking whether the modification of network dynamics after training could be beneficial for the persistence of the learned architecture compared with the random firing case. We reasoned that structured spontaneous activity ( Fig. 2d ) could consolidate the learned assembly structure, in line with proposals that link memory stability to reactivation during sleep or quiet wakefulness [40] . We therefore compared the trained recurrent network with a hypothetical non-recurrent network without structured spontaneous activity. Both networks began with the same initial trained weight matrix and exhibited the same firing rates (see Methods). However, in the non-recurrent network, synaptic plasticity modified the weight matrix depending on neurons’ spike times, but excitatory spikes did not cause excitatory postsynaptic potentials (EPSPs) in postsynaptic targets ( Fig. 4a ). Therefore, excitatory inputs were purely external and uncorrelated, which prevented coordinated assembly activation. We measured over a period of spontaneous activity in the two models. In the non-recurrent network, decayed faster than in the recurrent network with structured spontaneous activity ( Fig. 4b , compare black and yellow curves), despite the fact that neurons fired at the same rates in both networks. This suggests that the particular timing of assembly activation during structured spontaneous activity prevents degradation of learned network connectivity. 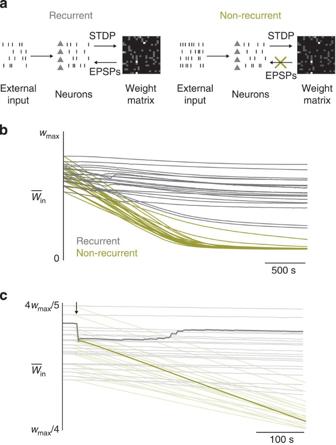Figure 4: Stability of trained architecture. (a) Schematic of recurrent and non-recurrent networks. In both networks, neurons fire leading to STDP that modifies the weight matrix. In the non-recurrent network, recurrent excitatory postsynaptic potentials (EPSPs) that would be caused by excitatory neuron spiking are blocked. (b) Average synaptic weight within assembliesduring spontaneous activity after training for the two networks. (c) Dynamics ofin response to a perturbation that reducedfor one assembly (solid lines) att=15 s (arrow). Results are shown for both the recurrent and non-recurrent network. Figure 4: Stability of trained architecture. ( a ) Schematic of recurrent and non-recurrent networks. In both networks, neurons fire leading to STDP that modifies the weight matrix. In the non-recurrent network, recurrent excitatory postsynaptic potentials (EPSPs) that would be caused by excitatory neuron spiking are blocked. ( b ) Average synaptic weight within assemblies during spontaneous activity after training for the two networks. ( c ) Dynamics of in response to a perturbation that reduced for one assembly (solid lines) at t =15 s (arrow). Results are shown for both the recurrent and non-recurrent network. Full size image To further probe the effect of structured spontaneous activity, we perturbed , reducing it by 10% for one assembly, and analysed the resulting dynamics. After the perturbation, increased for that assembly, showing that structured spontaneous activity can retrain a network if its architecture is weakly disrupted ( Fig. 4c , black curve). This was not true for the non-recurrent network ( Fig. 4c , yellow curve). Hence, structured spontaneous activity both lengthens the time scale over which a network can retain its learned connectivity and provides an error-correcting mechanism given disruptions of this connectivity. We note that this error-correcting mechanism provides a novel means by which a plastic network may maintain its learned architecture. Mechanisms that improve the stability of single synapses [22] , [38] may complement structured spontaneous activity in improving stability. However, such mechanisms, on their own, will not demonstrate recovery after a perturbation ( Fig. 4c ). This is because coordinated activation of entire assemblies during structured spontaneous activity is necessary for this recovery to occur. To verify that reached a steady state, we increased the speed of plasticity and simulated the network for 4,000 s. Indeed, most assemblies maintained potentiated values ( Supplementary Fig. 4 ). To verify that the rate of change of individual synaptic weights decreased during spontaneous activity as the network remained near a stable equilibrium, we plotted the summed instantaneous rate of change of weights across the network ( Supplementary Fig. 5 ). This quantity substantially decreased after training was complete, suggesting that the fluctuations in the connectivity matrix were indeed small. Finally, we also verified that our results were not dependent on the simulation time step [41] ( Supplementary Fig. 6 ). While we have focused mainly on the voltage-based excitatory STDP rule for clarity of exposition, we also tested our results using two other realistic plasticity rules: the triplet rule of Pfister and Gerstner [24] and the calcium-based rule of Graupner and Brunel [26] . All three rules exhibited a firing rate dependence of potentiation and depression, with high postsynaptic rates leading to strong potentiation ( Fig. 5a ). However, the calcium-based rule led to synaptic potentiation at sufficiently high presynaptic rates, even with low postsynaptic rates ( Fig. 5a , right). This implies that activation of assembly j will lead to potentiation of synapses from j to i in the absence of activation of i . This could potentially lead to interference between activated assemblies during the training protocol. Indeed, after training, the triplet and voltage-based rules behaved similarly, with spontaneous activity improving the stability of for most but not all assemblies, while the calcium-based rule behaved differently ( Fig. 5b ). For the calcium-based rule, increased for certain assemblies after training, suggesting that training was unable to fully potentiate synapses within assemblies. Furthermore, the calcium-based rule led to winner-take-all behaviour, with only certain assemblies remaining potentiated after training ( Fig. 5b,c , right). These results suggest that structured spontaneous activity improves stability for a variety of plasticity rules, but the details depend on the specific instantiation of the STDP rule. In particular, rules that potentiate when the presynaptic, but not postsynaptic, neuron fires at a high rate are likely to exhibit interference between assemblies during training. 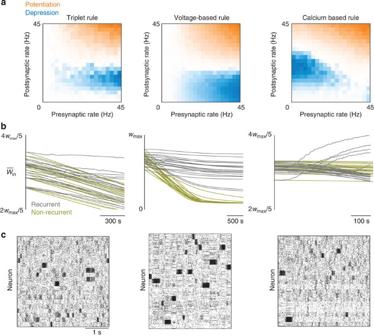Figure 5: Assembly formation with different STDP rules. (a) Schematic showing the average change in synaptic strength as a function of pre- and postsynaptic firing rate, assuming both neurons fire as Poisson processes. Results are shown for the triplet STDP rule of Pfister and Gerstner24(left), the voltage-based STDP rule of Clopathet al.25(center) and the calcium-based rule of Graupner and Brunel26(right). (b) Comparison between recurrent and non-recurrent networks as inFig. 4. Although the number of stored assemblies depends on the specific rule, structured spontaneous activity improves the stability of assemblies in all cases. (c) Structured spontaneous activity after training using the three rules. Figure 5: Assembly formation with different STDP rules. ( a ) Schematic showing the average change in synaptic strength as a function of pre- and postsynaptic firing rate, assuming both neurons fire as Poisson processes. Results are shown for the triplet STDP rule of Pfister and Gerstner [24] (left), the voltage-based STDP rule of Clopath et al. [25] (center) and the calcium-based rule of Graupner and Brunel [26] (right). ( b ) Comparison between recurrent and non-recurrent networks as in Fig. 4 . Although the number of stored assemblies depends on the specific rule, structured spontaneous activity improves the stability of assemblies in all cases. ( c ) Structured spontaneous activity after training using the three rules. Full size image Remapping architecture with novel stimuli We have shown that a set of stimulus patterns can be embedded in a recurrent network with STDP. How flexible is this network architecture? Can assemblies associated with novel stimulus sets be embedded in the network? We examined this question by defining a new set of 20 stimulus patterns and repeatedly presenting them to the network. We then compared for the new stimulus-defined assemblies and the old assemblies throughout this protocol. During this retraining protocol, increased for the new assemblies and decayed for the old assemblies ( Fig. 6a ). Fully potentiating the new set of assemblies required more stimulus presentations than the original training protocol, indicating that previously trained stimulus-specific assemblies can interfere with the formation of new ones. Retraining also shifted spontaneous activity. Prior to retraining, the original assemblies were activated during spontaneous activity ( Fig. 6b ). Afterwards, the new assemblies were activated ( Fig. 6c ). Given the stability of the trained assemblies ( Fig. 4 ) and these results, we conclude that the network architecture is stable to weak perturbations of its input statistics, but sufficiently strong changes in its inputs cause the network to reorganize itself. 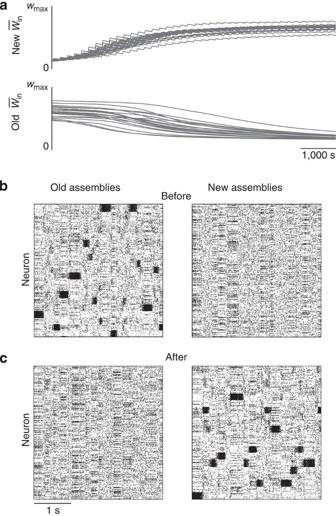Figure 6: Remapping of architecture with presentation of a new stimulus ensemble. (a) Average synaptic weight within assembliesfor neurons in the new set of assemblies (top) and the original set of assemblies (bottom), during repeated presentations of the new stimulus set. (b) Plot of network activity for rows arranged according to the original assemblies (left) and new assemblies (right). The activity is the same for both rasters, but the rows are permuted according to assembly membership. (c) Same asb, but after training on the new stimulus set. Figure 6: Remapping of architecture with presentation of a new stimulus ensemble. ( a ) Average synaptic weight within assemblies for neurons in the new set of assemblies (top) and the original set of assemblies (bottom), during repeated presentations of the new stimulus set. ( b ) Plot of network activity for rows arranged according to the original assemblies (left) and new assemblies (right). The activity is the same for both rasters, but the rows are permuted according to assembly membership. ( c ) Same as b , but after training on the new stimulus set. Full size image Mechanisms of stability and remapping in a reduced model The high dimensional and complex dynamics of our spiking network precluded a mathematically rigorous analysis of the dynamics of neuronal assemblies. In particular, it was not possible to formally reduce the dynamics of synaptic weights to a low-dimensional system whose stable states could be identified. In this section, we develop a simplified model of interacting neuronal populations that qualitatively reproduces the dynamics of assembly formation in the spiking network (see Supplementary Methods for a full descriptioin of the reduced model). We explore this model and show three core requirements for stable assembly structure: a firing rate-dependent plasticity rule, multistability in the firing rates of different assemblies and homeostasis. We considered two populations whose firing rates reflect the number of active neurons in the population at a given time (see Methods). Populations interacted according to a 2 × 2 excitatory synaptic weight matrix, as well as via global inhibition that was proportional to the total excitatory activity. We implemented a plasticity rule with a firing rate dependence similar to that of the spiking network ( Fig. 1a , bottom; see Methods). The change in the synaptic strength from population j to i was given by Δ W ij ∝ r j · r i ( r i − θ ), where r i is the firing rate of population i and θ is the threshold for potentiation. Strong potentiation therefore only occurred when both the postsynaptic and presynaptic firing rates, r i and r j , were large. When all synaptic weights were equal, both populations exhibited low levels of activity ( Fig. 7a , left). However, when recurrent excitation within populations 1 and 2 was strong ( W 11 = W 22 = w max ), the populations exhibited multistability and transitioned between low and high activity states, similar to the trained spiking network ( Fig. 7a , right). These different dynamics led to differential recruitment of plasticity. In particular, little plasticity was recruited when both populations had low rates, but the within-population weight W ii was strongly potentiated whenever population i was in a high activity state ( Fig. 7a , bottom). 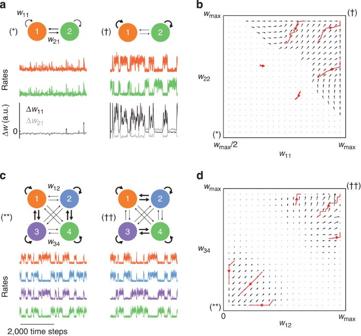Figure 7: Weight dynamics in the reduced model. (a) Two-population model in the untrained (left) and trained (right) states. Top: schematic illustrating weights. Thicker lines correspond to stronger weights. Middle: dynamics of population firing rates. Bottom: change in synaptic weights from population 1 onto itself (ΔW11) and population 1 to 2 (ΔW21) due to the rate fluctuations in the middle subpanel. (b) Vector field showing the weight dynamics forW11andW12. The top right is stable and corresponds to the right side ofa. Red trajectories correspond to individual simulations of the model. Fluctuations correspond to switching between distinct activity states; in the limit of infinitely slow learning, the trajectories would approach their steady state smoothly. (c) Similar toabut for the four-population model. Left: state in which populations (1,3) and populations (2,4) form a strongly connected assembly. Right: state in which populations (1,2) and populations (3,4) form a strongly connected assembly. (d) Vector field for the four-population model showing the weight dynamics forW12andW34. The bottom left corresponds to the left side ofc, and the top right corresponds to the right side ofc. Figure 7: Weight dynamics in the reduced model. ( a ) Two-population model in the untrained (left) and trained (right) states. Top: schematic illustrating weights. Thicker lines correspond to stronger weights. Middle: dynamics of population firing rates. Bottom: change in synaptic weights from population 1 onto itself (Δ W 11 ) and population 1 to 2 (Δ W 21 ) due to the rate fluctuations in the middle subpanel. ( b ) Vector field showing the weight dynamics for W 11 and W 12 . The top right is stable and corresponds to the right side of a . Red trajectories correspond to individual simulations of the model. Fluctuations correspond to switching between distinct activity states; in the limit of infinitely slow learning, the trajectories would approach their steady state smoothly. ( c ) Similar to a but for the four-population model. Left: state in which populations (1,3) and populations (2,4) form a strongly connected assembly. Right: state in which populations (1,2) and populations (3,4) form a strongly connected assembly. ( d ) Vector field for the four-population model showing the weight dynamics for W 12 and W 34 . The bottom left corresponds to the left side of c , and the top right corresponds to the right side of c . Full size image Similar to the spiking model, we assumed that each row of the 2 × 2 matrix defining the weights for the two populations summed to a constant (homeostatic synaptic normalization; W 11 + W 12 = W 22 + W 21 = w max ). This led to competition between the synapses onto each population. This feature allowed us to reduce the four-dimensional dynamics of the weights to a two-dimensional plane of W 11 and W 22 , the strength of the synaptic weight within each of the two populations. Further, since synaptic plasticity occurred on a time scale that is much slower than the stochastic activity of the population dynamics, we applied standard mathematical techniques from dynamical systems theory to derive the phase portrait for the synaptic weights ( Supplementary Methods ). Specifically, to determine the stability of any fixed points of W ij , we computed the vector field d W 11 /d t and d W 22 /d t for each location in the W 11 and W 22 planes (black arrows in Fig. 7d ). When both W ii were not potentiated, the network had only one stable activity level, and W ii did not change substantially ( Fig. 7a , left and Fig. 7b , bottom left). But when the W ii were sufficiently large, the system exhibited structured spontaneous activity and activation of populations drove the W ii to w max , their fully potentiated value ( Fig. 7a , right and Fig. 7b , top right). Thus, the model illustrated that when W ii is potentiated, structured spontaneous activity appears and causes W ii to approach w max . This dynamic makes the assembly structure ( W 11 = W 22 = w max ) stable to small fluctuations in W ij . Next, we extended the model to study the effects of remapping. We defined a four-population model in which each population was half the size of the two-population case, so that pairs of populations could together form assemblies with identical dynamics to Fig. 7a . When populations 1 and 3 were strongly connected and populations 2 and 4 were strongly connected, each pair (1,3) and (2,4) formed an assembly that underwent correlated fluctuations ( Fig. 7c , left). Further, if the connectivity was changed such that the pairs (1,2) and (3,4) were strongly connected, the new pairs underwent correlated fluctuations ( Fig. 7c , right). We examined the dynamics of the synaptic weights in the subspace spanned by W 12 and W 34 (see Methods). We found that both the (1,3) and (2,4) pairing ( Fig. 7c , left and Fig. 7d , bottom left) and the (1,2) and (3,4) pairing ( Fig. 7c , right and Fig. 7d , top right) were stable weight configurations. The model therefore shows that learned synaptic weight matrices can be stabilized by structured spontaneous activity, and that there may be multiple such stable weight matrices. As the number of possible combinations of subpopulations that can form assemblies increases, the number of stable weight matrices will grow exponentially. In total, our simplified model recapitulated the formation and remapping of stable assemblies that was the central result from the spiking model network. Our analysis identified the core requirements to be rate-dependent plasticity with potentiation reserved for high pre- and postsynaptic activity, coupled with bistable firing rate dynamics. Furthermore, the simplicity of the model suggests that the results of the spiking model did not critically depend on the exact choice of the spiking model neuron or synaptic dynamics. We note, however, that the simplified model is not formally derived from the spiking network, and therefore does not rigorously establish the stability of the spiking network. Spike statistics before and after training We have investigated the mechanisms that cause spiking network’s connectivity to reorganize due to input. Next, we quantify the resulting changes in spike train statistics. We examined the responses of neurons to the new set of stimulus patterns ( Fig. 6 ) before and after training on those patterns. This allowed us to make predictions about spontaneous and evoked dynamics before and after training. We first considered evoked firing rates. Consistent with increased recurrent connectivity, the gain of stimulated neurons was higher for trained versus untrained inputs ( Fig. 8a ). In addition to amplification, structured excitatory connectivity is often proposed as a mechanism for pattern completion [42] . To test whether the network could perform pattern completion, we presented stimuli that targeted half of the neurons in an assembly. We then compared firing rates of stimulated and non-stimulated neurons in targeted assemblies to baseline firing rates. Before training, stimulated neurons fired at increased rates, but non-stimulated neurons within a stimulated assembly fired at baseline levels ( Fig. 8b ). After training, both stimulated and non-stimulated neurons had increased firing rates. Hence, the presence of a stimulus could be read out from neurons that did not directly receive it through feedforward projections, as long as they were part of the corresponding assembly. 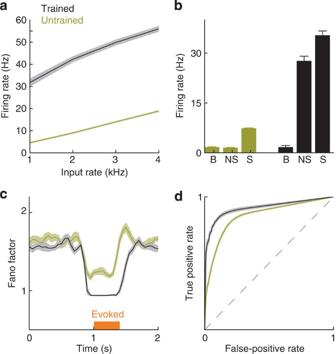Figure 8: Changes in evoked spike statistics after training on a new stimulus ensemble. (a) Average evoked firing rate in stimulated neurons as a function of stimulus strength, defined here as the change in the firing rate of the external excitatory input to stimulated neurons. All error bars denote s.e.m. across different stimuli. (b) Pattern completion before and after training. Average firing rates are shown in baseline spontaneous conditions (b), for non-stimulated neurons within a stimulated assembly (NS) and for stimulated neurons (S). (c) Fano factor as a function of time for all excitatory neurons. Evoked stimulation interval is denoted by the orange bar. Fano factor was computed using the mean-matching techniques presented in Churchlandet al.3(d) Average receiver-operating characteristic (ROC) curve for detecting the presence of a stimulus using the spike count of single neurons in the first 200 ms after stimulus onset. Figure 8: Changes in evoked spike statistics after training on a new stimulus ensemble. ( a ) Average evoked firing rate in stimulated neurons as a function of stimulus strength, defined here as the change in the firing rate of the external excitatory input to stimulated neurons. All error bars denote s.e.m. across different stimuli. ( b ) Pattern completion before and after training. Average firing rates are shown in baseline spontaneous conditions ( b ), for non-stimulated neurons within a stimulated assembly (NS) and for stimulated neurons (S). ( c ) Fano factor as a function of time for all excitatory neurons. Evoked stimulation interval is denoted by the orange bar. Fano factor was computed using the mean-matching techniques presented in Churchland et al. [3] ( d ) Average receiver-operating characteristic (ROC) curve for detecting the presence of a stimulus using the spike count of single neurons in the first 200 ms after stimulus onset. Full size image We also examined trial-to-trial variability of excitatory neurons in the network. We computed the Fano factor of spike counts in 100-ms windows over repeated stimulus presentations. Stimulation caused a reduction in Fano factor as is frequently observed in cortex [3] ( Fig. 8b ). This reduction was due to the suppression of spontaneous fluctuations by the stimulus [18] , [43] . The magnitude of this reduction was greater for trained versus untrained stimuli ( Fig. 8c ). This combination of decreased trial-to-trial variability and increased gain ( Fig. 8a ) suggests that training improved the reliability of stimulus representation. To test this, we attempted to detect the presence of a stimulus using the spike count of single neurons in 200-ms intervals after stimulus onset. The resulting receiver-operating characteristic curve was higher after training ( Fig. 8d ). Hence, training led to a measurable improvement in stimulus encoding, even at the single-neuron level. We also quantified collective activity using the spike count correlation between neuron pairs measured in 100-ms windows across trials. On average, correlations during spontaneous activity were near zero consistent with a balanced asynchronous state [17] ( Fig. 9a ). However, neuron pairs in the same assembly had positive average spontaneous spike count correlation after training ( Fig. 9b ). This correlation reflected collective fluctuations due to structured spontaneous activity. Notably, the contribution of these positive correlations was suppressed when the network was stimulated, with greater suppression for trained stimuli ( Fig. 9c ). We conclude that, after training, networks exhibit collective spontaneous fluctuations consistent with their previous inputs. However, when external input is applied, these fluctuations are suppressed and reliable responses are produced. 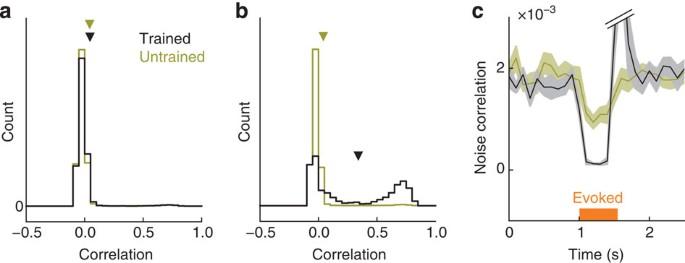Figure 9: Spike train co-variability before and after training. (a) Distribution of correlation coefficients during spontaneous activity for excitatory neuron pairs. Triangles denote means of distributions. (b) Same asafor neurons that shared membership in at least one assembly. (c) Average spontaneous spike count correlation as a function of time for all excitatory neurons. Evoked stimulation interval is denoted by the orange bar. Shaded region denotes s.e.m. across different stimuli. Figure 9: Spike train co-variability before and after training. ( a ) Distribution of correlation coefficients during spontaneous activity for excitatory neuron pairs. Triangles denote means of distributions. ( b ) Same as a for neurons that shared membership in at least one assembly. ( c ) Average spontaneous spike count correlation as a function of time for all excitatory neurons. Evoked stimulation interval is denoted by the orange bar. Shaded region denotes s.e.m. across different stimuli. Full size image We have explored how realistic synaptic plasticity rules combined with homeostatic mechanisms allow stable neuronal assemblies to form in balanced networks. The presence of these assemblies leads to spontaneous dynamics that reflect past stimuli. Previous studies have often neglected the influence of spontaneous dynamics on the stability of network architectures [15] , [22] , [25] . However, recent work showing large fluctuations in spontaneous spiking activity, similar in magnitude [44] and temporal patterning [2] to evoked states, challenges the validity of this assumption. We specifically investigated the interaction of ongoing synaptic plasticity with spontaneous dynamics, showing that spontaneous fluctuations can consolidate learned assemblies, rather than dissolving them. Clearly identifying neuronal assemblies is difficult because accessing a large fraction of the connections in a local circuit is experimentally challenging, although some progress has been made [45] . Our model, however, makes predictions that can be tested with single neurons or pairs ( Figs 8 and 9 ). One prediction, that recurrent connectivity is responsible for a large proportion of stimulus-tuned excitatory input, is consistent with findings from visual and auditory cortex that tuned recurrent excitation amplifies responses to thalamic input [46] , [47] , [48] . The fact that these responses are associated with slow dynamics [18] is also consistent with results from auditory cortex, suggesting that recurrent excitation prolongs response duration [48] . Taken together, our results are consistent with a picture of sensory cortex in which specific connectivity between functionally related neurons strongly influences cortical processing [49] . Experimental studies have demonstrated that spike train statistics can be modified by training or stimulus application. In our model, the formation of neuronal assemblies led to an increase in gain and reduction in trial-to-trial variability. Consistent with this, repeated presentation of an auditory stimulus increases gain and reduces variability of evoked membrane responses in auditory cortex [13] . An increase in firing rate and decrease in variability in neurons in prefrontal cortex was also found after training on a working-memory task [50] . Our network also makes predictions about spike train co-variability. Structured spontaneous activity leads to increased correlations for neurons with similar stimulus preference, as is commonly reported [8] , [9] . Further, because connectivity is related to stimulus preference in our network, this implies that neurons that share strong connections have higher correlations ( Fig. 9b ). This is consistent with findings from visual cortex showing noise correlations are higher for connected pairs [14] . While assembly dynamics have been studied previously, our model is the first to include balance, realistic STDP and stability of learned architecture after training. Amit and Brunel [21] did not explicitly model potentiation, instead assuming within-assembly synapses were selectively potentiated and then studying the resulting dynamics. Mongillo et al. [22] implemented plasticity, but assembly stability was due to bistability in synaptic weights owing to cellular mechanisms, as opposed to the network mechanisms presented in our work. Morrison et al. [23] implemented STDP without homeostatic mechanisms, and found that network dynamics were unstable. Further, none of these attractor studies examined the dynamics of networks with rich spontaneous dynamics including assembly reactivation. We show that, in fact, spontaneous dynamics can improve the stability of learned architectures ( Fig. 4 ), a feature lacking in models that obtain stability through synaptic mechanisms [22] , [38] . Izhikevich et al. [19] considered large, but non-balanced networks with extremely low (0.1%) connection probability, finding that neuronal assemblies randomly formed, but only persisted transiently. Finally, Brea et al. [51] examined learning in networks of Poisson neurons, showing that sequences could be learned with a specific learning rule that is similar to those studied in our manuscript. However, noisy sequences led to degradation of connectivity during spontaneous dynamics, as the stability mechanisms discussed in our study ( Fig. 4 ) were not present. Prior literature has proposed that reactivation of hippocampal neuronal ensembles is crucial for memory consolidation [40] . Computational models have argued that such reactivation can be beneficial for memory stability [27] , [28] . In these studies, connectivity perturbations were due to the formation of new associative memories. In contrast, we consider stability in the face of ongoing cortical spontaneous activity, which has proven difficult for stable models of cortical plasticity [23] , [34] , [35] . In both cases, reactivation is beneficial for memory stability. Our results suggest that, even in the absence of new learned associations, reactivation may prevent random firing from degrading learned connectivity. Further, cortical trial-to-trial variability permits reactivation without hippocampal input. Memory systems must contend with the ‘stability–plasticity dilemma,’ the fact that improving the stability of existing associations leads to difficulty in learning new associations. This is clearly visible in our model, as small perturbations of connectivity died out ( Fig. 4c ) while larger ones led to reorganization ( Fig. 6 ). Further work is necessary to determine what mechanisms precisely determine the region of stability for a given connectivity. Possible mechanisms that may promote plasticity for relevant inputs include neuromodulators that manipulate synaptic plasticity and signal for novelty [52] or feedforward iSTDP that biases responses towards novel stimuli [30] . We have shown that homeostatic regulation of firing rates in the form of iSTDP is crucial for robust training of the network ( Fig. 3 ). We do not claim that this particular form of plasticity is necessary, but rather that regulation of the average firing rate is likely important for maintaining stable activity patterns. Firing rate-modulated scaling of total excitatory input weight, for example, could accomplish similar effects. Indeed, miniature excitatory postsynaptic current sizes and firing rates increase following sensory deprivation that initially decreases visual cortex activity [53] . Previous theoretical studies have shown that homeosynaptic scaling can be beneficial for heterogeneous working-memory circuits, similar to how iSTDP prevents winner-take-all dynamics [36] ( Fig. 3 ). Our network also relied on heterosynaptic competition, which maintained a neuron’s total excitatory synaptic input, and bounds on synaptic strength. Heterosynaptic competition has been studied experimentally and in model networks [29] , [37] , [54] . In a previous computational model, normalization of both presynaptic and postsynaptic weights along with a simple STDP rule led to the spontaneous development of feedforward chains [37] . Our model, in contrast, includes a dependence of STDP on firing rate and fewer constraints on synaptic weights, leading to qualitatively different dynamics. Bounds on synaptic strength were also necessary to curb the instrinsic instability of excitatory STDP. Without them, strong stimuli could cause assemblies’ recurrent weights to increase without limit, or, conversely, parts of the network to become completely disconnected. Such pathological behaviour has been observed in previous models of balanced excitatory–inhibitory networks with STDP that lacked the homeostatic mechanisms in our study [23] . Previous studies have investigated whether STDP is capable of embedding trajectories in neural activity space into recurrent networks [55] , [56] . In these studies, STDP that depended only on spike timing was combined with homeostatic rules to produce networks that respond to inputs with stereotyped trajectories. These networks tend to produce effectively feedforward connectivity matrices [37] , [56] , in contrast to the the overlapping assemblies of our study. Such assemblies, along with the concordant increase in the likelihood of strong reciprocal coupling between pyramidal neurons, are observed in experimental data [45] , [57] . This difference is likely due to our incorporation of firing rate-dependent STDP, which allows for the formation of Hebbian assemblies. We also explicitly investigated the persistence of the learned connectivity during spontaneous activity, a feature that is lacking in these studies. Future work should reconcile these prior investigations with firing rate-dependent STDP and rich spontaneous activity. We made several assumptions on plasticity in our network. For simplicity and due to lack of experimental studies, we did not model plasticity of synapses onto inhibitory neurons. We also assumed feedforward inputs to neurons were fixed during training. In development, thalamic input specificity occurs before recurrent specificity is established [15] , supporting this assumption. In our network, training causes a shift from responses being driven in a purely feedforward manner to one in which recurrent excitation is dominant ( Fig. 8a ). This is reminiscent of predictive coding theories, in which higher regions predict the activity in lower regions and feedforward connections serve primarily to transmit errors in this prediction [58] . We expect that plasticity of feedforward projections would also support this type of computation, with feedforward inhibitory plasticity suppressing the transmission of redundant stimuli. Our synaptic time constants were faster than those estimated from experiments to reduce simulation time [25] . The time scale separation argument in our reduced model (see Methods) suggests that our results will hold for slower weight changes, as does the fact that different learning speeds led to similar results ( Supplementary Fig. 4 ). The primary requirement for stable learning is that homeostatic mechanisms must be sufficiently fast relative to the excitatory STDP to prevent runaway dynamics in the latter. In the limit of very slow inhibitory STDP, the network will be unable to solve the problem of winner-take-all dynamics ( Fig. 3 ). This result is consistent with a recent study that showed fast homeostatic mechanisms are necessary to stabilize excitatory STDP in recurrent networks [34] . A critical aspect of our model was the dependence of potentiation and depression on the firing rate of the postsynaptic neuron ( Fig. 1a , bottom). Such dependence has been shown experimentally and is a feature of multiple biophysically motivated STDP rules [24] , [25] , [26] , [33] , all of which reproduced the results of this study ( Fig. 5 ). Unlike previous studies in which spike timing was the only determinant of synaptic changes, firing rate, not spike timing, was the most important quantity in our network. Indeed, our reduced model captured many features of the spiking network using plasticity similar to rate-based Bienenstock-Cooper-Munro rules [59] , and all three STDP rules had qualitatively similar rate dependences. However, while we have shown that neuronal assemblies constitute stable configurations of the synaptic weights for our system, we have not shown that they are the only ones. Other structures, such as feedforward chains, may also be stabilized by STDP. Relating biophysically motivated plasticity rules to the stable weight configurations they can support remains an open area of inquiry. Membrane potential dynamics The model network consisted of N E excitatory (E) and N I inhibitory (I) neurons. Throughout, we will denote population (E or I) with superscripts and neuron index (1 through N E/I ) by subscripts. The equation for the voltage dynamics of neuron i in population X was: Parameter values are summarized in Table 1 . Dynamics are consistent with Clopath et al. [25] Excitatory units were modelled as exponential integrate-and-fire neurons with an adaptation current and adaptive threshold [31] , [32] . Inhibitory units were modelled as simple non-adapting integrate-and-fire neurons . The dynamics of the neuronal threshold for excitatory neurons, , were given by: Table 1 Parameters for neuronal membrane dynamics. Full size table When neuron i spiked due to its voltage diverging (in simulation, determined by voltage exceeding 20 mV), its potential was reset to V re and clamped for an absolute refractory period of τ abs . If it was excitatory, its threshold was set to V T + A T . For inhibitory neurons, at all times. We denote the spike train of neuron i in population X as , where are the times when the neuron spiked and δ is the Dirac delta function. The adaptation current for excitatory neuron i , , was given by: When excitatory neuron i spiked, was increased by b w . Dynamics of synaptic conductances Connections occurred with probability p , and the strength of a connection from neuron j in population Y to neuron i in population X was denoted . If a connection did not exist, . Recurrent excitatory connection weights were bounded by and , while weights from inhibitory to excitatory neurons were bounded by and . J IE and J II were fixed and constant for all connected i , j . The total excitatory or inhibitory conductance of neuron i in population X was given by: where Y ε ( E , I ), F Y ( t ) is the synaptic kernel for input from population Y , and * denotes convolution. Synaptic kernels were given by a difference of exponentials: for t positive. In addition to recurrent input, neurons also received external excitatory input in the form of a spike train , which was an independent homogeneous Poisson process for each neuron with rate . This input may be interpreted as the sum of 1,000 independent excitatory presynaptic neurons, each with a firing rate . For external excitatory input, the synaptic strength was set to the minimim recurrent synaptic strength . Neurons did not receive external inhibitory input . Parameters were chosen such that a fully potentiated excitatory or inhibitory synapse onto an excitatory neuron caused a postsynaptic potential of ~2.5 mV if all other inputs were blocked. Synapses were implemented with a delay between 0 and 1.5 ms using the techniques of Mattia and Giudice [60] with a resolution of 0.1 ms. Parameter values can be found in Table 2 . Table 2 Parameters for recurrent coupling. Full size table Excitatory synaptic plasticity We implemented a voltage-based STDP rule [25] that modified within the bounded range . Furthermore, we imposed a homeostatic normalization of the total excitatory synaptic weights that a neuron received by scaling each row of every 20 ms to maintain a constant row sum [36] , [37] . This was accomplished by subtracting a constant amount from each nonzero entry in the row: , where is the number of nonzero entries. The dynamics of the synapse from excitatory neuron j to excitatory neuron i were given by: where R is a linear-rectifying function ( R ( x )=0 if x <0, R ( x )= x otherwise), and represent the membrane voltage low-pass filtered with time constants τ u and τ υ , respectively, and represents the spike train low-pass filtered with time constant τ x . Parameter values can be found in Table 3 . Table 3 Parameters for excitatory synaptic plasticity. Full size table Inhibitory synaptic plasticity We implemented an inhibitory STDP rule [30] that modified within the bounded range . Weight changes depended on , which represents the spike train low-pass filtered with time constant τ y . Upon a spike from either the presynaptic or postsynaptic neuron, the weight was modified according to the following: The rate r 0 represents the target firing rate to which the inhibitory plasticity attempts to balance the postsynaptic neuron. During unstimulated conditions, neurons fired on average less frequently than their target rate due to synaptic bounds (mean of 1.7 Hz rather than 3 Hz; Supplementary Fig. 3 ), allowing the system to exhibit a distribution of firing rates because of the variability in the connectivity matrix. Parameter values can be found in Table 4 . Table 4 Parameters for inhibitory synaptic plasticity. Full size table Stimulation protocols For training ( Fig. 2 ), each stimulus i =1…20 was activated sequentially for a period of 1 s, with 3-s gaps in between stimulus presentations. This was repeated until each stimulus had been repeated 20 times. For retraining ( Fig. 6 ), each stimulus was presented 80 times. During training, stimuli increased by 8 kHz. These simulations began with a 10-s period without STDP to allow transients to die out. To probe the dependence of Fano factor and correlation before and after training ( Figs 8 and 9 ), we used a weaker stimulus, with a duration of 500 ms and an increase in of 2 kHz. These simulations were repeated 50 times for each of the 10 stimuli to assess trial-to-trial variability. We disabled STDP for these short protocols. For the non-recurrent network ( Fig. 4a,b ), we chose the inhibitory STDP target firing rate for each neuron to be equal to its spontaneous firing rate in the trained system and removed synaptic bounds for inhibitory STDP. We also increased by 4 kHz and by 2 kHz to compensate for the loss of recurrent excitation. We then allowed the system to run for 200 s for firing rates to reach their target values before activating excitatory STDP. This allowed for a matched firing rate comparison between the two networks. Simulations were performed using code written in Python, C++ and Julia implementing Euler integration with a time step of 0.1 ms. Code implementing the model written in Julia is available at http://www.ugcs.caltech.edu/~alk/code/alk_formation_2014.zip . Other plasticity rules For the triplet-based rule ( Fig. 5 , left), the following parameters were used (following the notation of Pfister and Gerstner [24] ): τ + =16.8 ms, τ _=33.7 ms, τ x =101 ms, τ y =125 ms, , , , . For the calcium-based rule ( Fig. 5 , right), the following parameters were used (following the notation of Graupner and Brunel [26] ): γ p =7.25, γ d =3.31, θ p =1.3, θ d =1, τ Ca =22.7 ms, C pre =0.56, C post =1.24. Reduced model Our reduced model ( Fig. 7 ) consisted of neuronal populations defined similarly to Bressloff [61] . Briefly, the activity of population i was given by n i , which represented the number of neurons in an ‘active’ state. Transitions from a state of n i active neurons to n i ±1 active neurons occurred with rates , making n i a birth–death process. The transition rates were given by and , where n is the vector of active neurons for each population. Here N is an abstract system-size parameter; we note that it is not equal to the maximum of n i , which can exceed N . We therefore define x = n / N , which can have entries greater than 1. As N →∞, the dynamics of x reduce to the Wilson–Cowan equations: [61] . The activation function was given by: For sufficiently large W ii , this nonlinear activation function yields bistability in the corresponding Wilson–Cowan system as N →∞ ( Fig. 7a , right). The excitatory weight matrix W ij was constrained to have a constant row sum, , in the same manner as the spiking simulations. Entries in W ij were bounded by 0 and w max and evolved according to where η =0.001 is the learning rate and θ =1.8 is the potentiation threshold. For the two-population model, w max =1, w inh =0.2 and N =16. For the four-population model, w max =1/2, w inh =0.1 and N =8 so that pairs of populations could form a single population identical to the two-population case. Bressloff [61] presented techniques to analyse the rate of transitions for a single population x i from a low activity state x i = x L to a high activity state x i = x H separated by a saddle point x 0 . Defining and , the rate of transitions from a state x L/H is given by: We extended this framework to the case of multiple populations to compute the vector field of Fig. 7b . Given a W ij , we first numerically calculated the solutions { x *} to the deterministic Wilson–Cowan equations and determined which were stable. We then calculated transition rates between stable solutions using equation (9) by assuming only one population i transitioned at a time and other populations’ activities remained fixed during the transition, , and then afterwards settled to their new local equilibrium values. These transition rates yielded a Markov process over metastable states of the system with equilibrium density P ( x *). Assuming η was small so a time scale separation could be performed, the expected change in W ij was calculated as: The vector field of Fig. 7d was numerically estimated. Simulations of the reduced system were done using the Gillespie algorithm. Further details are given in Supplementary Methods . How to cite this article: Litwin–Kumar, A. and Doiron, B. Formation and maintenance of neuronal assemblies through synaptic plasticity. Nat. Commun. 5:5319 doi: 10.1038/ncomms6319 (2014).